Multiparametric atomic force microscopy imaging of single bacteriophages extruding from living bacteria Force-distance (FD) curve-based atomic force microscopy is a valuable tool to simultaneously image the structure and map the biophysical properties of biological samples at the nanoscale. Traditionally, FD-based atomic force microscopy has been severely limited by its poor temporal and lateral resolutions. Here we report the use of advanced FD-based technology combined with biochemically sensitive tips to image filamentous bacteriophages extruding from living bacteria at unprecedented speed and resolution. Directly correlated multiparametric images of the structure, adhesion and elasticity of infected bacteria demonstrate that the sites of assembly and extrusion localize at the bacterial septum in the form of soft nanodomains surrounded by stiff cell wall material. The quantitative nano-bio-imaging method presented here offers a wealth of opportunities for mapping the physical properties and molecular interactions of complex biosystems, from viruses to tissues. Introduced in the 1990s, force-distance (FD) curve-based atomic force microscopy (AFM) [1] , [2] , [3] , [4] enables researchers to correlate structural images of complex biological systems with quantitative maps of their biophysical properties. The principle is to record spatially resolved FD curves across the biological sample [3] , [5] . From each curve, a given property (for example, adhesion or elasticity) is extracted, quantified and displayed as grey (or coloured) pixel, the brightness of which reflects the magnitude of the measured property. In doing so, spatially resolved maps of sample properties and interactions are produced. Until recently, the low speed and poor spatial resolution of this method have severely hampered its widespread use in biology. However, recent progress in FD-based AFM has enabled the circumvention of these limitations, and has provided a unique means to record directly correlated, multiparametric images of the structure, adhesion and elasticity of biological systems at (near) molecular resolution and at the speed of conventional topographic imaging (for a recent review, see Dufrêne et al. [6] ). This newer technology has already been used to simultaneously image the structure and the biophysical properties of complex specimens, including human keratinocytes [7] , diatoms [8] , yeasts [9] , lipid phases [10] , membrane proteins [11] , [12] , [13] , virus capsids [14] and pathological neurofibrils [15] . In the membrane protein context, the method was applied to map quantitatively the flexibility of individual membrane proteins in their native, folded state at unprecedented submolecular resolution and to correlate protein flexibility with crystal structure [13] . In other studies, the technique enabled structural mapping of the deformation, adhesion, energy dissipation and elasticity of native proteins at a resolution of a few nanometres [11] , and quantification of the electrostatic field and potential generated by transmembrane protein pores at subnanometer resolution [12] . Although valuable, these experiments lack biochemical specificity, that is, they cannot identify nor force probe specific constituents (for example, a given receptor) in complex, heterogeneous systems (for example, living cells). Hence, the quantitative multiparametric imaging of specific biochemical sites using advanced FD-based AFM remains very challenging. Here, we combine the use of advanced FD-based AFM with specific microscope tips to simultaneously image the structure of heterogeneous biological systems and quantitatively map their adhesion and mechanical properties. As a prototype complex biological sample, we investigate the extrusion of individual filamentous bacteriophages from the surface of living bacteria. Filamentous bacteriophages (Φ), such as fd, f1 and M13, are 880 nm long and 6 nm-wide structures with a circular single-stranded DNA (ssDNA) genome, that are able to infect a variety of Gram-negative bacteria such as Escherischia coli ( Fig. 1a ) [16] , [17] , [18] . The ssDNA encodes three classes of proteins, that is, replication (pII, pX and pV), morphogenetic (pI, pIV and pXI) and structural (pVIII, pIII, pVI, pVII and pIX) proteins ( Fig. 1a ). The constitutive proteins are anchored in the inner membrane and incorporated into the virion using a specialized assembly site working as an aqueous channel where the inner and outer membranes are in close contact ( Fig. 1b ) [19] , [20] . Initiation of assembly starts with the addition of pIX and pVII on the packaging signal. Then, pV, which collapses the ssDNA into a flexible rod in the cytosol, is progressively replaced by the major coat protein pVIII as the phage particle is extruded from the outer membrane ( Fig. 1b ). Once the ssDNA is coated by pVIII, pIII and pVI are added to the late extremity of the virion and the phage is released from the cell, a process that can be blocked by the deletion of pIII (ΦpIIId) [17] , [18] , [21] . Although phage replication and assembly have been extensively studied in vitro , the cellular localization of the sites of phage assembly and release are poorly understood, owing to the paucity of high-resolution imaging techniques. To address this issue, in this work E. coli bacteria infected by His-tagged Φ particles are imaged using advanced FD-based AFM with biochemically sensitive tips, that is, tips functionalized with Ni 2+ -NTA groups. Directly correlated multiparametric images of the structure, adhesion and elasticity of infected bacteria enable us to demonstrate that the sites of the assembly machinery localize at the bacterial septum in the form of soft nanodomains surrounded by stiff cell wall material. This biospecific multiparametric imaging method offers unprecedented possibilities to quantify and spatially map the multiple biophysical properties of complex biomolecular and cellular systems in physiological conditions. 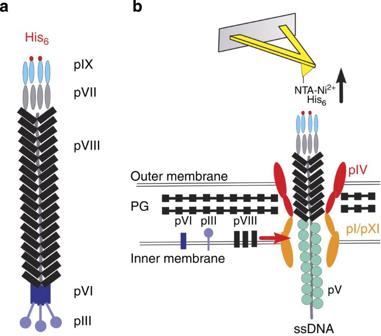Figure 1: Probing single bacteriophages using AFM with biochemically sensitive tips. (a) Filamentous bacteriophages were genetically engineered to display His-tag on their pIX tail. (b) Single phages assembled in and escaping from the bacterial cell wall were detected via their His-pIX tail using an AFM tip modified with Ni2+-NTA groups. Shown in the cartoon are the main components of the assembly machinery (see text for details). Figure 1: Probing single bacteriophages using AFM with biochemically sensitive tips. ( a ) Filamentous bacteriophages were genetically engineered to display His-tag on their pIX tail. ( b ) Single phages assembled in and escaping from the bacterial cell wall were detected via their His-pIX tail using an AFM tip modified with Ni 2+ -NTA groups. Shown in the cartoon are the main components of the assembly machinery (see text for details). Full size image Fluorescence imaging of infected bacteria We first analysed the expression of pIX-His-tagged bacteriophages (f1 filamentous bacteriophages [22] ; Φwt) in E. coli bacteria using fluorescence microscopy, following labelling with Ni 2+ -NTA fluorescent conjugates ( Fig. 2 ). Phage production occurred predominantly near the septum and the poles of the bacteria ( Fig. 2a,d ). We compared the behaviour of wt phages with that of mutant phages in which the pIII gene had been inactived by sequence frameshift (ΦpIIId). pIII proteins are required for infectivity and stability of the particles. Bacteria infected with ΦpIIId produce particles that are not released into the medium but remain associated at the surface in the assembly machinery [23] . Bacteria infected with ΦpIIId were homogeneously labelled ( Fig. 2b,e ), confirming that phages that lack pIII stayed anchored into the cell wall. Labelling specificity was confirmed by showing that non-infected bacteria were not fluorescent ( Fig. 2c,f ). 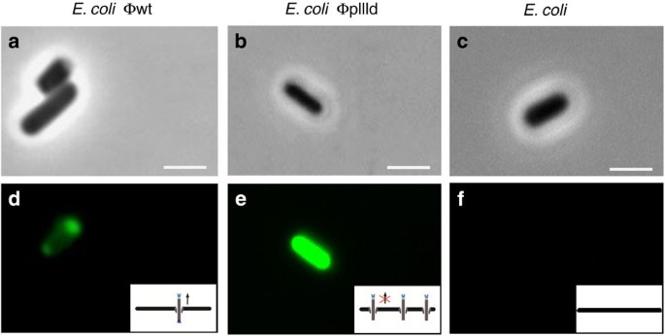Figure 2: Fluorescence imaging of bacteria infected by bacteriophages. Phase (a–c) and fluorescence (d–f) images ofE. colicells infected by Φwt (a,d) or by ΦpIIId particles lacking pIII (b,e) and of non-infectedE. colicells (c,f), following labelling with Ni2+-NTA fluorescent conjugates. Scale bar 2 μm. Figure 2: Fluorescence imaging of bacteria infected by bacteriophages. Phase ( a – c ) and fluorescence ( d – f ) images of E. coli cells infected by Φwt ( a , d ) or by ΦpIIId particles lacking pIII ( b , e ) and of non-infected E. coli cells ( c , f ), following labelling with Ni 2+ -NTA fluorescent conjugates. Scale bar 2 μm. Full size image FD-based AFM visualizes single bacteriophages We then imaged E. coli bacteria infected by Φwt using FD-based AFM with Ni 2+ -NTA-terminated tips ( Fig. 3 ). While structural images revealed a smooth, featureless surface ( Fig. 3a ), directly correlated adhesion maps were highly contrasted, adhesion events being primarily detected in the septum or polar regions ( Fig. 3b ). In these regions, the adhesion events corresponded to an apparent surface density of 617±294 sites μm − 2 ( n =1,700 FD curves from 17 different maps from three independent experiments). As FD curves are recorded at frequencies three orders of magnitudes higher than in classical FD-based AFM, the imaging speed and resolution are greatly increased (~8 min for a 256 × 256 pixel image versus ~80 min for a 64 × 64 pixel image). From high magnification views ( Fig. 3b , lower inset), we estimate that the resolution of our adhesion images is a few nanometres. Increasing the resolution further, although technically feasible, would have no sense in this study as this would lead to detecting the same sites multiple times. We note that structural and adhesion maps were obtained at a maximum applied force of 1 nN, yielding an indentation of ~50 nm. The contrast of our structural images ( Fig. 3 ) was similar to that obtained in conventional contact mode, and was not altered by the applied force (within the 0.1–1 nN range). 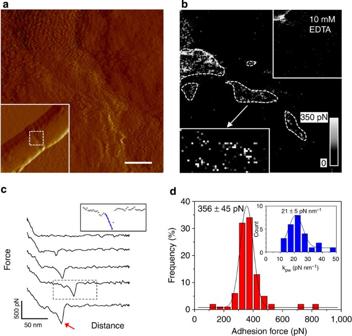Figure 3: Imaging the extrusion of single bacteriophages from living bacteria using FD curve-based AFM. (a) FD-based AFM structural image (scale bar, 200 nm; error signal; inset: low-resolution image; the high-resolution image was recorded in the dashed square) and (b) directly correlated adhesion map (upper inset: same experiment in the presence of EDTA; lower inset: enlarged view of an adhesive area) of anE. colicell infected with Φwt particles recorded in PBS with a Ni2+-NTA tip. (c) Representative FD curves. The red arrow on the bottom curve indicates the maximum adhesion force corresponding to the rupture of the His–Ni2+-NTA bond. The linear shape of the adhesion force peaks (inset: linear fit) indicates that the phage–cell wall complex behaves as a Hookean spring. (d) Histogram of adhesion forces (n=500 adhesion events from three independent experiments, that is, using three different tip preparations and three independent cultures). The inset shows the distribution of the spring constant values associated with the phage–cell wall complex (n=500). Figure 3: Imaging the extrusion of single bacteriophages from living bacteria using FD curve-based AFM. ( a ) FD-based AFM structural image (scale bar, 200 nm; error signal; inset: low-resolution image; the high-resolution image was recorded in the dashed square) and ( b ) directly correlated adhesion map (upper inset: same experiment in the presence of EDTA; lower inset: enlarged view of an adhesive area) of an E. coli cell infected with Φwt particles recorded in PBS with a Ni 2+ -NTA tip. ( c ) Representative FD curves. The red arrow on the bottom curve indicates the maximum adhesion force corresponding to the rupture of the His–Ni 2+ -NTA bond. The linear shape of the adhesion force peaks (inset: linear fit) indicates that the phage–cell wall complex behaves as a Hookean spring. ( d ) Histogram of adhesion forces ( n =500 adhesion events from three independent experiments, that is, using three different tip preparations and three independent cultures). The inset shows the distribution of the spring constant values associated with the phage–cell wall complex ( n =500). Full size image We believe that the measured adhesion events correspond to the specific detection of single phage particles for several reasons. First, non-infected bacteria imaged with the same method showed essentially no adhesion events ( Fig. 4i ); second, treatment of infected bacteria with 10 mM EDTA led to a substantial decrease of adhesion frequency, indicating that NTA tips lacking Ni 2+ are no longer able to detect His-tagged particles ( Fig. 3b , upper inset); third, bacteria infected with ΦpIIId were massively labelled ( Fig. 4g ), confirming that phages lacking pIII remain surface-associated; and fourth, adhesive FD curves showed well-defined adhesion force peaks ( Fig. 3c , see red arrow on lower curve) of 356±45 pN (mean±s.d., n =500 adhesive events from three independent experiments) ( Fig. 3d ). These adhesion events correspond to the rupture of the bond between the Ni 2+ -NTA tip and a single His-tagged bacteriophage since they are in the range of the force expected for single Ni 2+ -NTA–His interactions at the loading rate that we used (~10 7 pN s −1 ) (refs 24 , 25 , 26 ). 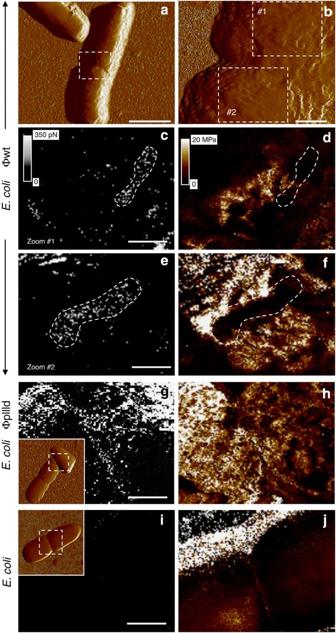Figure 4: Bacteriophage extrusion localizes into soft nanodomains. (a) Low- and (b) high-resolution FD-based AFM structural images (error signal) ofE. colicells infected by Φwt particles recorded in PBS with Ni2+-NTA AFM tips. Scale bar ina, 2 μm. Scale bar inb, 300 nm. (c,e,g,i) Directly correlated adhesion maps and (d,f,h,j) elasticity maps (z-scale shows Young’s modulus values) ofE. colicells infected by Φwt (c–f) or by ΦpIIId particles lacking pIII (g,h) and of non-infectedE. colicells (i,j). Scale bars are: (c) 150 nm, (e) 150 nm, (g) 500 nm and (i) 300 nm. Imagesc,d,eandfcorrespond to the zoomed areas shown in panelb. The insets in panelsgandiare the low-resolution topography images on which imagesg–jwere recorded (see dashed squares). The dashed lines inc–femphasize the organization of the bacteriophages into soft nanodomains surrounded by stiff material. Similar results were obtained in seven independent experiments (that is, experiments using seven different tip preparations and seven independent cultures) forE. colicells infected by Φwt particles (see alsoFig. 5), in five independent experiments forE. colicells infected by ΦpIIId particles and in three independent experiments for non-infectedE. colicells. Figure 4: Bacteriophage extrusion localizes into soft nanodomains. ( a ) Low- and ( b ) high-resolution FD-based AFM structural images (error signal) of E. coli cells infected by Φwt particles recorded in PBS with Ni 2+ -NTA AFM tips. Scale bar in a , 2 μm. Scale bar in b , 300 nm. ( c , e , g , i ) Directly correlated adhesion maps and ( d , f , h , j ) elasticity maps (z-scale shows Young’s modulus values) of E. coli cells infected by Φwt ( c – f ) or by ΦpIIId particles lacking pIII ( g , h ) and of non-infected E. coli cells ( i , j ). Scale bars are: ( c ) 150 nm, ( e ) 150 nm, ( g ) 500 nm and ( i ) 300 nm. Images c , d , e and f correspond to the zoomed areas shown in panel b . The insets in panels g and i are the low-resolution topography images on which images g – j were recorded (see dashed squares). The dashed lines in c – f emphasize the organization of the bacteriophages into soft nanodomains surrounded by stiff material. Similar results were obtained in seven independent experiments (that is, experiments using seven different tip preparations and seven independent cultures) for E. coli cells infected by Φwt particles (see also Fig. 5 ), in five independent experiments for E. coli cells infected by ΦpIIId particles and in three independent experiments for non-infected E. coli cells. Full size image Interestingly, most adhesion events were not randomly distributed but organized into nanodomains, 190±258 nm 2 in size ( n =105 domains from 17 different maps from five independent experiments) ( Fig. 3b ; clusters are highlighted by dashed lines). The nanoscale organization of Φwt is reminiscent of the behaviour of lytic bacteriophages shown to form discrete 50–200 nm lytic holes at the septum and occasionally at the poles [27] . We suggest that the assembly machinery can only be located near the septum (and the poles), where peptidoglycan is synthesized. Indeed, pI, pIV and pXI are known to form a channel across the whole bacterial cell wall breaking the peptidoglycan layer [28] . As no enzymes encoded by the phage are able to disrupt peptidoglycan, we expect that the assembly machinery should be integrated at the sites of peptidoglycan synthesis, that is, where cell division takes place. Nanomechanics of the phage–cell wall complex How do single phages respond to mechanical force? FD curves recorded for Φwt were well-described by a linear fit, rather than by a worm-like chain model, which is characteristic of a Hookean behaviour ( Fig. 3c , inset). Considering the spring constant of the AFM cantilever ( k c ) and the slope ( s ) of the linear portion of the raw deflection versus piezo displacement curves, the apparent spring constant of the phage–cell wall complex ( k pw ) is given by k pw =( k c × s )/(1−s)=21±5 pN nm –1 (mean±s.d., n =500 adhesive curves from five independent experiments) ( Fig. 3d , inset). As the bacteriophage is a non-deformable filament [29] , [30] , k pw primarily reflects the bacterial cell wall stiffness. Supporting this view, our measured values are close to the bacterial spring constant measured for E. coli [31] . We note that FD curves recorded for bacteria infected with ΦpIIId particles also showed linear force behaviours with similar spring constant values. Notably, the linear force peaks that we observed here are very different from those reported earlier for Φwt particles that were simply adsorbed on solid surfaces [30] . Pulling on adsorbed phages yielded non-linear force peaks that were preceded by extended elongation events, up to several hundreds nanometres, reflecting the progressive desorption and straightening of the phages into extended orientations. Such force signatures were never observed here, leading us to conclude that the detected Φwt particles were actively extruded from the bacteria and not simply adsorbed on the cell surface in a non-specific manner. Consistent with this, similar linear force peaks were observed for bacteria infected with ΦpIIId particles. Bacteriophage extrusion localizes into soft nanodomains Next, we used multiparametric imaging to correlate the structural, adhesion and mechanical properties of infected bacteria ( Figs 4 and 5 ). Correlated adhesion maps ( Figs 4c,e and 5a,c,e ) and elasticity (Young’s modulus) maps ( Figs 4d,f and 5b,d,f ) obtained for bacteria infected by Φwt revealed that bacteriophages were preferentially detected in soft regions (0.6±0.2 MPa; n =100 curves from three independent experiments), somewhat similar to the softness of native bacteria (1.0±0.3 MPa; n =100 curves from three independent experiments), and generally surrounded by much stiffer cell wall properties (11.4±5.9 MPa; n =100 curves from three independent experiments). Such quantitative correlations were found in multiple independent experiments ( Figs 4 and 5 ). Cells infected by ΦpIIId ( Fig. 4g,h ) showed a dense distribution of phages in the adhesion image, that was correlated with heterogeneous, complex cell wall properties, that is, soft spots surrounded by a stiff matrix. By contrast, non-infected cells ( Fig. 4i,j ) showed no phage detection and homogeneously soft properties (1.0±0.3 MPa; n =100 curves from three independent experiments) that are typical of those reported for native E. coli bacteria [32] . The differences in local mechanical properties that we unravelled here may be biologically relevant. Because the assembly machinery of the phages is localized near the septum, that is, where peptidoglycan synthesis takes place, we expected that these nanodomains may interfere with peptidoglycan assembly, leading to the accumulation of newly formed cell wall material around these sites. 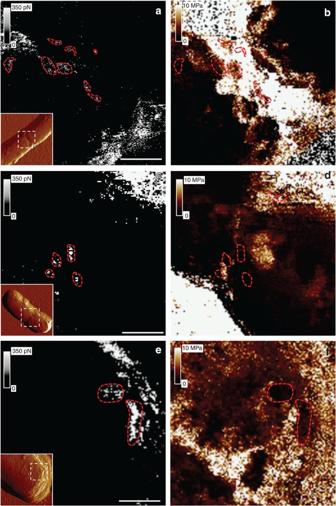Figure 5: Simultaneous imaging of the adhesion and elasticity of infected bacteria. (a,c,e) Adhesion maps and (b,d,f) directly correlated elasticity maps recorded by FD-based AFM with Ni2+-NTA AFM tips onE. colicells infected by Φwt. The insets in panelsa,c,eare the low-resolution structural images on which adhesion and elasticity images were recorded. The dashed lines emphasize the organization of the bacteriophages into soft nanodomains surrounded by stiff material. Scale bars are: (a) 250 nm, (c) 250 nm and (e) 125 nm. Figure 5: Simultaneous imaging of the adhesion and elasticity of infected bacteria. ( a , c , e ) Adhesion maps and ( b , d , f ) directly correlated elasticity maps recorded by FD-based AFM with Ni 2+ -NTA AFM tips on E. coli cells infected by Φwt. The insets in panels a , c , e are the low-resolution structural images on which adhesion and elasticity images were recorded. The dashed lines emphasize the organization of the bacteriophages into soft nanodomains surrounded by stiff material. Scale bars are: ( a ) 250 nm, ( c ) 250 nm and ( e ) 125 nm. Full size image A crucial challenge in current biological sciences is to characterize the structure, physical properties and interactions of cellular and biomolecular systems under physiological conditions. Our experiments demonstrate that advanced FD-based AFM combined with biochemically sensitive tips represents a powerful multiparametric characterization platform for the simultaneous imaging of the structural and biophysical properties of complex biosystems. To the best of our knowledge, this is the first time that correlated structural, adhesion and elasticity images of complex biological samples are recorded at high temporal and spatial resolutions, and with biochemical specificity. The speed (few minutes) and resolution (few nanometres) are similar to those of classical topographic imaging, thus exceeding markedly the performances of conventional FD-based AFM. In addition to mapping single-receptor sites and sample elasticity, individual FD curves can also provide quantitative information on the nanomechanics of the stretched receptors. Using this method, we provide the first direct visualization of the assembly machinery of bacteriophages on live cells, revealing that it localizes near the septum in the form of soft nanodomains surrounded by stiffer cell wall material. Applicable to a wide variety of complex biological systems, from viruses to tissues, this quantitative, biospecific imaging method offers new opportunities for understanding crucial biological processes and functions. Bacterial strains E. coli TG1: F′ [ traD36 proAB + lacI q lacZΔM15 ] supE thi-1 Δ(lac-proAB) Δ(mcrB-hsdSM)5, (r K − m K − ) was from Invitrogen. His-tag pIX phages were produced by the strain TG1 harbouring the phagemid pUPP9His/Tag [30] and already infected by the helper phage R408, a derivative of the filamentous phage f1 (ref. 22 ). His-tagged pIX pIIId phages (pIII deficient) were produced by the strain TG1, transformed with the pUPP9His/Tag phagemid and infected by a filamentous phage in which the pIII gene is inactivated by a frameshift in an open reading frame inserted between the sequences encoding the signal peptide and the mature pIII [33] . Fluorescence microscopy E. coli bacteria were washed three times by centrifugation (2,000 g for 5 min) in phosphate-buffered saline (PBS), incubated in 50 μg ml −1 of Ni 2+ -NTA-Atto conjugates for 1 h in the dark at 20 °C and washed two times with PBS. Images were acquired with a Zeiss Axio Observer Z1 equipped with a Hamamatsu camera C10600. AFM measurements AFM measurements were performed at 20 °C in buffered solutions (PBS, pH 7.4) with a Bioscope Catalyst AFM (Bruker AXS Corporation, Santa Barbara, CA), using the newly developed peak force tapping mode (PeakForce-Quantitative Nano-Mechanics). Cells were immobilized onto high-molecular weight polyethyleneimine-coated glass petri dishes, as described elsewhere [34] . Bacterial cultures (200 μl) were centrifuged three times at 2,000 g for 5 min and resuspended in PBS. The cell suspension was deposited onto polyethyleneimine-coated glass for 1 h and then extensively rinsed with PBS. V-shaped Scan Asyst fluid cantilevers (Bruker AXS Corporation) with a spring constant of 0.45–0.77 N m −1 were coated by electron beam thermal evaporation with a 5-nm-thick Cr layer followed by a 30-nm-thick Au layer. Gold-coated cantilevers were immersed overnight in ethanol containing 0.1 mM of NTA-terminated (10%) and triethylene glycol-terminated (90%) alkanethiols (ProChimia, Poland), rinsed with ethanol and then further incubated with a 40-mM solution of Ni 2+ . Multiparametric images were recorded at 256 pixels × 256 pixels with a driving frequency of 0.25 kHz, and an applied force of 1 nN. Cantilever spring constant and sensitivity were calibrated before and after each experiment. Data processing was performed using the commercial Nanoscope Analysis software (Bruker AXS Corporation). Young’s moduli were calculated using the Sneddon model for a conical tip. How to cite this article: Alsteens, D. Multiparametric atomic force microscopy imaging of single bacteriophages extruding from living bacteria. Nat. Commun. 4:2926 doi: 10.1038/ncomms3926 (2013).